Self-assembly of amorphous calcium carbonate microlens arrays Biological materials are often based on simple constituents and grown by the principle of self-assembly under ambient conditions. In particular, biomineralization approaches exploit efficient pathways of inorganic material synthesis. There is still a large gap between the complexity of natural systems and the practical utilization of bioinspired formation mechanisms. Here we describe a simple self-assembly route leading to a CaCO 3 microlens array, somewhat reminiscent of the brittlestars' microlenses, with uniform size and focal length, by using a minimum number of components and equipment at ambient conditions. The formation mechanism of the amorphous CaCO 3 microlens arrays was elucidated by confocal Raman spectroscopic imaging to be a two-step growth process mediated by the organic surfactant. CaCO 3 microlens arrays are easy to fabricate, biocompatible and functional in amorphous or more stable crystalline forms. This shows that advanced optical materials can be generated by a simple mineral precipitation. Natural materials often grow by biologically controlled self-assembly processes under ambient conditions [1] , [2] . Despite using easily accessible materials only, they often show remarkable functional properties. For example, biominerals in many skeletons are strong and have a crucial role in supporting and/or protecting the bodies of living organisms. Some biominerals also function as optical devices in organisms. This is seen in glass sponges and brittlestars [3] , [4] , for example, where optical fibres and microlenses show exceptional optical performances originating from optimized biomineral shape or crystal orientation. Biomineralization has been widely studied to first understand how inorganic materials are produced under the control of organic molecules in nature and second to apply this knowledge in synthetic systems [5] , [6] , [7] , [8] , [9] . There have been reports on the synthetic fabrication of CaCO 3 structures, which mimic biominerals via templating; such as the replica of the sea urchin skeletal plate [10] , [11] , the micropatterned single calcite crystal [12] and periodic optical nanostructures of inverse opal [13] . These studies have demonstrated that biomineral structures could be reconstructed by using a biomimetic mineralization approach and showed how to utilize the most representative characteristics of biomineralization, namely, amorphous precursor pathways and templates [14] , [15] , [16] . These synthetic procedures remain restricted to small sample sizes, are still very complex and also require further steps for preparing or removing biological or artificial templates. Various fabrication methods combined with lithographic techniques have been demonstrated to be practical for the synthesis of microlens arrays [17] , [18] , [19] , [20] , [21] , [22] . However, these techniques are limited to the fabrication of microlens arrays on flat substrates and require multiple steps, such as baking, developing and etching. Furthermore, the aforementioned approaches yield to microlens arrays made of organic materials with comparatively low refractive indices. However, it is often desirable to have a high refractive index and short focal lengths. This can be achieved using inorganic materials. Here we show how these microlens arrays can be synthesized by a simple mineral precipitation process without any template and at ambient conditions. In this work, we prepared arrays of CaCO 3 microlenses with uniform size and focal length by using a saturated calcium solution and CO 2 in air, together with a widely used surfactant as the base materials. To understand the formation mechanism of the microlens structures, confocal Raman spectroscopic imaging was carried out to characterize the three main components: carbonate, water and organic. The role of the organic molecules, acting as a surface-active and structure-directing agent, is discussed and we draw conclusions on how the uniformity of the structures is achieved. Furthermore, this article reports on the biocompatibility as well as the optical properties of the microlens arrays at the micro- and macroscopic scale. Synthesis and formation of the CaCO 3 microlens arrays CaCO 3 precipitates start to form and agglomerate at the interface of air and saturated Ca(OH) 2 solution right after the solution reacts with CO 2 in air. The synthesis process is schematically described in Fig. 1a . This surface aggregation goes on for 15–20 min with Brownian motion ( Supplementary Movie 1 ). The scanning electron microscopy (SEM) images in Fig. 1b,c clearly show the nanometre-sized CaCO 3 precipitates adhered to the agglomerates, as indicated by white arrows. The agglomerates attain a quasi-hemispherical shape and diameter of up to 2.7 μm within 2 min ( Fig. 1b,c ). The CaCO 3 agglomerates are also formed in the absence of surfactant or monolayers, although the morphology is not uniform in this case ( Supplementary Fig. S1a ). The role of the surfactant, polysorbate 20 (non-ionic, or Tween 20, PS 20), composed of fatty acid esters of polyoxyethylene sorbitan, is to regulate the growth of CaCO 3 agglomerates into a uniform size and shape ( Supplementary Fig. S1 ). PS 20 molecules have adsorbed onto the CaCO 3 precipitates and agglomerates at the early stage of growth based on a time-dependent surface tension measurement, as depicted in Fig. 1a . In these measurements, the surface tension of water containing 10 μM of PS 20 ranged from 40 to 55 mN m −1 ( Supplementary Fig. S2 ), demonstrating that the surfactant was located at the air–water interface. However, the surface tension of Ca(OH) 2 solution with the same concentration of the surfactant was close to that of pure water, 70 mN m −1 , indicating that only a few surfactant molecules were located at the air–solution interface. This clearly demonstrates that most of the surfactant must adsorb onto the precipitates and the quasi-hemispherical agglomerates. Indeed, considering the critical micelle concentration of PS 20 (80 μM at 21 °C), hydrophilic groups of the non-ionic surfactant are likely to be adsorbed on the hydrophilic surface of CaCO 3 (ref. 23 ). 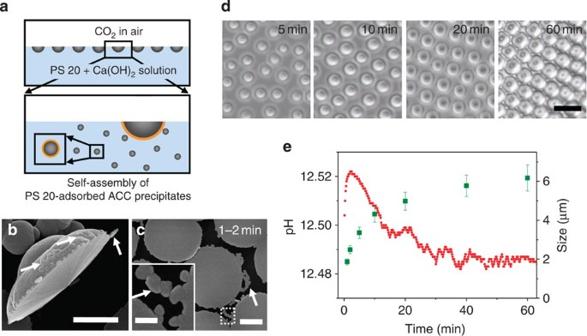Figure 1: Formation of CaCO3microlens array. (a) Schematic illustration for the formation of CaCO3microlens array. (b,c) SEM images of CaCO3agglomerates after 1–2 min of reaction. The scale bars are 1 μm. The inset ofcis a magnified image of the white dotted box. The scale bar is 200 nm. White arrows indicate the nanometre-sized CaCO3precipitates. (d)In situoptical microscopy images observed on the surface of Ca(OH)2solution versus reaction time. The scale bar is 10 μm. (e) The changes of both pH (red dot) in Ca(OH)2solution and averaged size (green rectangle) of CaCO3microlens with standard deviation plotted versus time (statistics from size measurement of 150 microlenses for each time point, 50 microlenses from each of three different samples). Figure 1: Formation of CaCO 3 microlens array. ( a ) Schematic illustration for the formation of CaCO 3 microlens array. ( b , c ) SEM images of CaCO 3 agglomerates after 1–2 min of reaction. The scale bars are 1 μm. The inset of c is a magnified image of the white dotted box. The scale bar is 200 nm. White arrows indicate the nanometre-sized CaCO 3 precipitates. ( d ) In situ optical microscopy images observed on the surface of Ca(OH) 2 solution versus reaction time. The scale bar is 10 μm. ( e ) The changes of both pH (red dot) in Ca(OH) 2 solution and averaged size (green rectangle) of CaCO 3 microlens with standard deviation plotted versus time (statistics from size measurement of 150 microlenses for each time point, 50 microlenses from each of three different samples). Full size image As the CaCO 3 agglomerates grow, the floating agglomerates self-assemble to form a close packed two-dimensional array and are linked together by further growth. The growth of these agglomerates was monitored in real time by optical microscopy in transmission mode for 1 h, and the images obtained at different reaction times are shown in Fig. 1d . The size of the CaCO 3 agglomerates and pH change of the solution plotted versus the reaction time is shown in Fig. 1e . The growth speed, estimated from the slope of the agglomerate size as a function of time ( Fig. 1e ), fits to the corresponding decrease in pH. As shown below, the proton concentration increases when carbonate ions are combined with Ca ions to form precipitates [24] : Ca 2+ +CO 2 +H 2 O→Ca 2+ +H 2 CO 3 →Ca 2+ +H + +HCO 3 − →Ca 2+ +2H + +CO 3 − →2H + +CaCO 3 . The morphology of CaCO 3 microlens arrays after 60 min of growth is represented by a hexagonally packed array of hemispherical structures of homogeneous size and shape ( Fig. 2a,b ). The microlenses are connected to each other forming a film, as shown by the SEM image of sectionally cut CaCO 3 microlens arrays by focused ion beam milling ( Fig. 2b ). 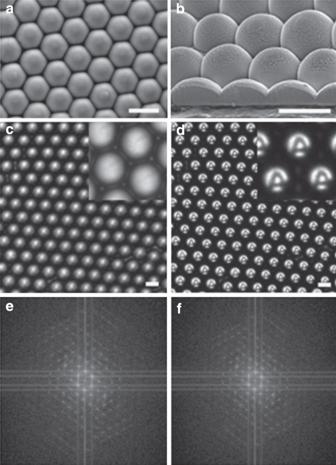Figure 2: Morphology and optical properties of the CaCO3microlens array. (a) SEM image of the homogeneous and well-ordered CaCO3microlens array from top view. (b) SEM image of cross-sectioned microlens array from 52° tilted view. The microlens array was etched by using focused ion beam with Ga ion beam. The bright layer on the surface of the microlens is the Pt coating, the surface without Pt coating was damaged by the ion beam and shows roughness as a result. The microlens structures were connected with each other. (c,d) Optical microscopy images of CaCO3microlens array and inversely projected 'A' array, respectively. The magnified images are shown in each inset. (e,f) The Fourier transformed images fromcandd, respectively. All the scale bars are 5 μm. Figure 2: Morphology and optical properties of the CaCO 3 microlens array. ( a ) SEM image of the homogeneous and well-ordered CaCO 3 microlens array from top view. ( b ) SEM image of cross-sectioned microlens array from 52° tilted view. The microlens array was etched by using focused ion beam with Ga ion beam. The bright layer on the surface of the microlens is the Pt coating, the surface without Pt coating was damaged by the ion beam and shows roughness as a result. The microlens structures were connected with each other. ( c , d ) Optical microscopy images of CaCO 3 microlens array and inversely projected 'A' array, respectively. The magnified images are shown in each inset. ( e , f ) The Fourier transformed images from c and d , respectively. All the scale bars are 5 μm. Full size image Optical properties The microlenses are consistent in shape and exhibit homogenous optical properties across an entire array. Figure 2c is the optical transmission image of a microlens array. Figure 2d shows the multiple image of a single 'A' projected through the array of microlenses [25] . The projected 'A' image is 3.2 μm, which is 620 times smaller than the 2 mm object 'A'. The projected images of 'A' are uniform in size and shape, which indicates the uniformity of the structures and focal lengths of the microlenses. This was further confirmed by a Fourier transformation of the images Fig. 2c,d into Fig. 2e,f , respectively. The discrete dot patterns indicate that the repeating units in Fig. 2e,f are uniform and well ordered. The projected image of the 'A' array in Fig. 2d is not observed by optical microscopy under crossed polarization. In addition, the microlens array does not show any peaks in X-ray diffraction ( Supplementary Fig. S3 ), which means that it is composed of amorphous CaCO 3 (ACC). The ACC microlens array was crystallized into calcite by thermal heating over 300 °C ( Supplementary Fig. S3 ). The cross-polarized light microscopy image of the calcite microlens array shows birefringency ( Supplementary Fig. S4 ). The microlenses keep their shape after crystallization and the array still shows the projected images of 'A' even under cross-polarized light because of birefringence. The optical image obtained with the ACC lenses ( Fig. 2d ) is clearer than the optical image with crystalline lenses ( Supplementary Fig. S4b ), probably because of the birefringence of the calcite microlenses. This characteristic is not observed with biomineralized single calcite microlens arrays in the brittlestar, Ophiocoma wendtii [4] , [22] . This is because, in the case of brittlestar, the non-birefringent optical axis is perpendicular to the microlens arrays. The light path through an ACC microlens array and the focal length are characterized by confocal microscopy as shown in Fig. 3 (ref. 26 ). 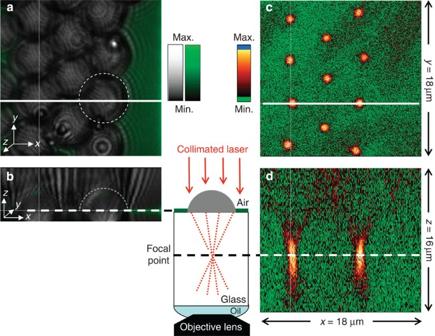Figure 3: Characterization of the focal length of the microlens array. (a,b) Fluorescence and brightfield confocal images of the microlens array and (c,d) characterization of the focal length of the microlenses. (a)x–yplane image of the microlens array resulting from the overlay of the brightfield image (grey scale) showing the microlenses, and the fluorescence image (green) showing the fluorescently labelled chitosan coating of the microscope coverslip. The brightfield and fluorescence images were recorded simultaneously by illumination/excitation at 488 nm and collection at 488 and 530 nm (± 25 nm), respectively. The circular dashed line shows the localization of a microlens in the array. (b)x–zplane image that represents a cross-section through a stack of images taken at different depths in the sample. The plane shown corresponds to the position indicated by a solid white line on imagea. The thick dashed line is aligned with the fluorescence from the chitosan coating and corresponds to the glass surface. The thin dashed line (semicircle) indicates the microlens curved surface. (c)x–yplane image of the light from a collimated laser beam (650±10 nm) focused by the microlenses, at a depth in the sample equal to their focal length. Imageccorresponds to the depth at which a dashed line on imagedhas been drawn. (d)x–zplane image of the light from a collimated laser beam (650±10 nm) focused by the microlenses. The image results from a cross-section taken through a stack of images recorded at different depth in the sample. The plane shown corresponds to the position indicated by a solid white line on imagea. The thin dashed vertical lines inaandb(candd, respectively) are a guide to the eye to match the images in thex-direction. The diagram in the middle of the figure shows a schematic of the confocal microscope with one microlens (grey filled semicircle) on a chitosan-coated (green line) cover glass (white box) and the beam path (red dotted lines). Figure 3c shows 11 spots corresponding to the light of a collimated laser beam focused at the back focal plane of the microlens array as shown in Fig. 3a . The beam waists at the focal plane of the microlenses were uniform in size and smaller than 1.2 μm (measured at full width at 1/e 2 ). The x – z plane images in Fig. 3b,d show the position of the chitosan coating at the surface of the microlenses in contact with the microscope coverslip and the converging light path at the back plane of the microlenses, respectively. To calculate the focal length of the microlenses, we measured their thickness by atomic force microscopy line scans and the distance from the back plane of the microlenses and the focused point ( Supplementary Fig. S5 ). We measured a focal length of 7.2±0.3 μm. The focal length of the microlenses focusing in the glass coverslip was calculated using the relation, where R =3.1±0.2 μm is the radius of curvature calculated based on the geometry of 11 microlenses measured by atomic force microscopy line scans, and n glass and n ACC are refractive indices of glass (1.50) and ACC (1.58, taken from the measured value of 1.5791–1.5830 by Merten and group [27] ), respectively. Entering these parameters into equation (1), we find f =8.0±0.5 μm. Figure 3: Characterization of the focal length of the microlens array. ( a , b ) Fluorescence and brightfield confocal images of the microlens array and ( c , d ) characterization of the focal length of the microlenses. ( a ) x – y plane image of the microlens array resulting from the overlay of the brightfield image (grey scale) showing the microlenses, and the fluorescence image (green) showing the fluorescently labelled chitosan coating of the microscope coverslip. The brightfield and fluorescence images were recorded simultaneously by illumination/excitation at 488 nm and collection at 488 and 530 nm (± 25 nm), respectively. The circular dashed line shows the localization of a microlens in the array. ( b ) x – z plane image that represents a cross-section through a stack of images taken at different depths in the sample. The plane shown corresponds to the position indicated by a solid white line on image a . The thick dashed line is aligned with the fluorescence from the chitosan coating and corresponds to the glass surface. The thin dashed line (semicircle) indicates the microlens curved surface. ( c ) x – y plane image of the light from a collimated laser beam (650±10 nm) focused by the microlenses, at a depth in the sample equal to their focal length. Image c corresponds to the depth at which a dashed line on image d has been drawn. ( d ) x – z plane image of the light from a collimated laser beam (650±10 nm) focused by the microlenses. The image results from a cross-section taken through a stack of images recorded at different depth in the sample. The plane shown corresponds to the position indicated by a solid white line on image a . The thin dashed vertical lines in a and b ( c and d , respectively) are a guide to the eye to match the images in the x -direction. The diagram in the middle of the figure shows a schematic of the confocal microscope with one microlens (grey filled semicircle) on a chitosan-coated (green line) cover glass (white box) and the beam path (red dotted lines). Full size image Structural characterization by Raman spectroscopy The CaCO 3 microlenses show structural complexity as found by depth scans with confocal Raman spectroscopic imaging ( Fig. 4 ), revealing the distribution of carbonate, water and organic components. A schematic illustration of a depth scan is shown in Fig. 4a . 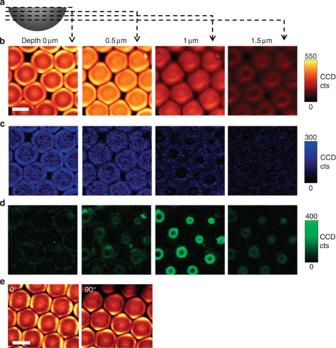Figure 4: Confocal Raman spectroscopic imaging of the CaCO3microlens array. (a) Schematic illustration of the depth scan. (b–d) Depth scanned Raman imaging obtained by integrating over the wavenumber ranges of (b) carbonate (1,040–1,125 cm−1), (c) water (3,000–3,500 cm−1) and (d) organic components (2,800–3,000 cm−1), respectively. The images in the same column indicate the same depth. (e) Raman imaging of carbonate at 0° and 90° polarization of incident laser light. All the scale bars are 5 μm. CCD cts, charge-coupled device counts. Figure 4b shows confocal Raman images of carbonate (spectral region 1,040–1,125 cm −1 ) at different depths. The Raman spectra in this band show the characteristics of ACC ( Supplementary Fig. S6 ). In the ACC, the band slightly shifts to lower wavenumbers and is characterized by a significant broadening (full-width at half-maximum 28 cm −1 in our experimental results), compared with that found in calcite [28] , [29] . However, the intensity of carbonate varies strongly through different z -section planes. In addition, at the depth positions from 0 to 0.5 μm, the Raman scattering of carbonate is higher at the edge than in the inner parts of the microlenses ( Fig. 4b ). This could be due to the preferential orientation of the carbonate units in the near-edge region of each microlens, as demonstrated by polarized Raman imaging with different polarization direction ( Fig. 4e ) [30] . The direction of the incident laser polarization was found to have no influence on the intensity of spectra in the inner part of the microlenses ( Supplementary Fig. S6 ). However, the upper/lower edges of the microlenses shows higher intensity with 90° polarization with respect to 0° and vice versa for the left/right edges ( Fig. 4e and Supplementary Fig. S6 ). Figure 4: Confocal Raman spectroscopic imaging of the CaCO 3 microlens array. ( a ) Schematic illustration of the depth scan. ( b – d ) Depth scanned Raman imaging obtained by integrating over the wavenumber ranges of ( b ) carbonate (1,040–1,125 cm −1 ), ( c ) water (3,000–3,500 cm −1 ) and ( d ) organic components (2,800–3,000 cm −1 ), respectively. The images in the same column indicate the same depth. ( e ) Raman imaging of carbonate at 0° and 90° polarization of incident laser light. All the scale bars are 5 μm. CCD cts, charge-coupled device counts. Full size image Confocal Raman imaging furthermore shows the molecular distribution of water and organic components in the microlens arrays ( Fig. 4c,d ). Thermogravimetric analysis gives the quantitative information that 1.46 wt% of organic is included in the hydrated ACC, which also contains about 1 mol of water ( Supplementary Fig. S7 ). The organic component is mainly distributed inside the microlenses at a depth of 1 μm ( Fig. 4d ). The water peak reduces in intensity at exactly the same position ( Fig. 4c ). It is noticeable that the organic rings are located inside the microlens structures with diameters of 2–3 μm, which means they were formed during the early stages of microlens formation (within 2 min, Fig. 1e ). This is consistent with the result of the surface tension measurement that most of the surfactant must be adsorbed on CaCO 3 precipitates and agglomerates right after the reaction starts ( Supplementary Fig. S2 ). We deduce a two-step growth of the ACC microlenses based on the observations of microlens-sizes as a function of time and on molecular detection by Raman imaging. The width of the anisotropic edge in Fig. 4e is 1–2 μm, which is similar to the grown size during the last 40–50 min in Fig. 1e . This is a very slow growth in comparison with the 4–5 μm of growth that occurs in the first 10–20 min. The slow growth at the edges of the microlenses could be explained by the formation from ion constituents or equivalent small molecules after the fast growth is obtained by aggregation of ACC nanometre-sized precipitates by Brownian collision. The distribution of organic matter, visible by the green ring in Fig. 4d , reflects the fact that the early precipitates agglomerate together with surfactant molecules to form the first nucleus of a microlens at the initial stage of growth at 1–2 min. The adsorbed surfactant is thought to have an essential role in the formation of the final CaCO 3 structures with uniform shape and size. Further growth of the microlenses occurs by the accretion of precipitates without organic components, which—at this stage—are already exhausted in the solution. It is notable that the complex inner structure of the microlenses (visible in Fig. 4 ) does not affect the optical images of the 'A's, as shown in Fig. 2d . Therefore, we deduce that the inclusion of the organic phase (1.46 wt% as determined by thermogravimetric analysis) does not distort the optical light path significantly. Moreover, the focal distance of the microlenses does not seem to be considerably influenced by the organic inclusions ( Fig. 3 ). The visualization of the complex structure in which organic components, amorphous and/or crystalline CaCO 3 phases coexist is not an easy task [8] , [14] , [31] , [32] , [33] . Aizenberg et al . [31] , [32] have shown the combination of the two CaCO 3 phases separated by an organic membrane in an ascidian skeleton by selective etching. In addition, several studies have reported how to visualize the distribution of organic components in synthetic or biogenic CaCO 3 matrices [8] , [33] . In the present work, Raman spectroscopic imaging successfully shows how the amorphous phase of CaCO 3 with preferential orientation of carbonates and organic matrix is distributed without destroying the mineral matrix. However, the organic–mineral interface and their interaction—in general being the hallmark of biomineralization or biomimetic mineralization [6] , [34] —remain to be further investigated in our system. One possible interpretation would be that the lipids of surfactant molecules stabilize the amorphous structure in the centre of the microlenses [16] , [32] . The carbonate groups are being more oriented in the outer parts of the microlenses, which might also be related with a directional guidance by the organic molecules forming a ring pattern. Indeed, the alkyl chain of self-assembly monolayers has been reported to be involved in the oriented growth of calcite [35] , [36] . The size of CaCO 3 microlens array films only depends on the area of the interface between precursor solution and air, which means there is basically no limitation for the fabrication of large film areas. 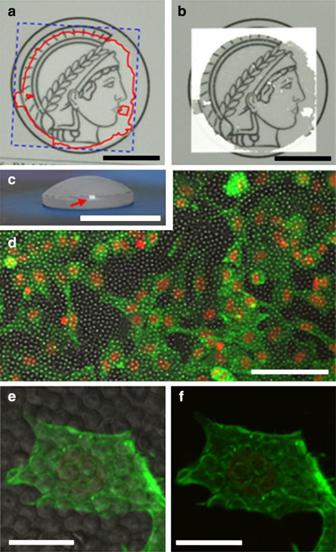Figure 5: CaCO3microlens arrays fixed on chitosan-coated substrates. (a,b) The pictures of the same CaCO3microlens array-chitosan composite film coated on a cover glass were taken at different angles, which shows the antireflecting effect of the composite film. (a) Blue dashed line and red solid line indicate the locations of the cover glass and the CaCO3microlens array, respectively. (b) The picture was taken at the right angle when the cover glass reflects incident light. Only the area where the CaCO3microlens array was coated keeps transparency. (c) The picture of the composite film coated on a convex quartz glass lens in the form of compound eye. The red arrow indicates the uncoated part, which reflects light. Scale bars ina–care 1 cm. (d) Overview of NIH3T3 fibroblast cell growth on the microlens array. Cells were stained with actin (green), and nucleus (red) with fluorescent dyes (overlay of fluorescent and phase contrast images). The scale bar is 100 μm. (e,f) Actin organization within the cell at higher magnification (e, overlay;f, green fluorescence). The scale bars are 20 μm. Figure 5 shows that CaCO 3 microlens arrays can be attached to gently curved surfaces as well as to flat ones on the centimetre-scale by using chitosan as glue. When the film of the CaCO 3 microlens array is coated on a cover glass, the repeated micron-sized convex structures prevent incident light from reflecting and keep the transparency as shown in Fig. 5a,b . This method can be used to coat microlens structures onto curved surfaces similar to that found on the moth eye ( Fig. 5c ) [37] , which is not possible with lithographic techniques [17] , [18] , [19] , [20] , [21] . These are effective antireflective lenses over the spectrum of visible light. Moreover, microlens arrays are compatible for cell attachment and growth as shown in Fig. 5d . Higher magnification on one individual cell, covering several tens of microlenses, shows the actin organization within the cell in response to the arrangement of the microlens array ( Fig. 5e,f ). Actin fibres are observed along the cell boundary and also around the microlens structures as the cell can feel the topography and adapt its cytoskeleton to the geometry of the microlens array [38] . This biocompatibility of the CaCO 3 material enables the presented microlens arrays to interact with a biological environment in a similar way as its archetype—the brittlestar. Figure 5: CaCO 3 microlens arrays fixed on chitosan-coated substrates. ( a , b ) The pictures of the same CaCO 3 microlens array-chitosan composite film coated on a cover glass were taken at different angles, which shows the antireflecting effect of the composite film. ( a ) Blue dashed line and red solid line indicate the locations of the cover glass and the CaCO 3 microlens array, respectively. ( b ) The picture was taken at the right angle when the cover glass reflects incident light. Only the area where the CaCO 3 microlens array was coated keeps transparency. ( c ) The picture of the composite film coated on a convex quartz glass lens in the form of compound eye. The red arrow indicates the uncoated part, which reflects light. Scale bars in a – c are 1 cm. ( d ) Overview of NIH3T3 fibroblast cell growth on the microlens array. Cells were stained with actin (green), and nucleus (red) with fluorescent dyes (overlay of fluorescent and phase contrast images). The scale bar is 100 μm. ( e , f ) Actin organization within the cell at higher magnification ( e , overlay; f , green fluorescence). The scale bars are 20 μm. Full size image In conclusion, we were able to show that highly ordered CaCO 3 microlens arrays with a specific focal length can be grown synthetically under ambient conditions by organic molecule controlled self-assembly of ACC precipitates. The formation mechanism is based on a two-step growth process, starting with a fast self-assembly of nanometre-sized precipitates followed by a retarded growth with oriented carbonate groups at the edge of the microlenses. The amphiphilic molecules have a crucial role at the very early stage of self-assembly and their arrangement is one of the prerequisites for the uniform hemispherical shape of the microlenses. In addition, the biocompatibility of the composite films consisting of biomineral microlenses and biopolymer will potentially enable the application for cell biology research combined with optics. In general, our findings further improve current capabilities to fabricate micrometre-scaled optical devices by using easily available materials and simple but efficient processing, and demonstrate that it is highly useful to consider biominerals as archetypes for the synthesis of advanced materials. Synthesis of CaCO 3 microlens arrays Ca(OH) 2 clear solution was prepared by dissolving 1 g of Ca(OH) 2 powder (Aldrich) in 100 ml millipore water, followed by complete sedimentation of a white substance after 3 days in a sealed media bottle. Calculated amounts of PS 20 (Aldrich) were added into the clear Ca(OH) 2 solution and stirred vigorously. A volume of 350 μl of precursor solution was dropped into each well of a 96 microplate, whose cover was left open in the atmosphere. After 1 h of reaction, a thin film of CaCO 3 microlens array was formed on the surface of the solution in each well. The film was skimmed off by using a microscope cover glass after adding 50–80 μl of water in each well and thereby the surface of solution with the film was raised over the top of the plate. The residual solution on the cover glass was soaked up by using lint-free tissue paper and dried in air. The convex side of the CaCO 3 microlens array was arranged towards the cover glass at this stage and the Raman characterization and the 'A' projection experiments were carried out as deposited. For SEM images, the CaCO 3 microlens arrays on a cover glass were transferred to a carbon tape allowing the curved surfaces to be investigated. The films of a CaCO 3 microlens array shown in Figs 3 and 5 were grown for 3 h in each well of 12-well plates filled with 5 ml of precursor solution. After the films were transferred to a cover glass and dried, they were attached on another cover glass or convex quartz glass lens (15 mm of focal length) coated with 2 wt% of chitosan solution in the same way described above, which was followed by drying under nitrogen. For the characterization of the light path through the microlens array and its focal length, the fluorescently labelled chitosan solution was used to detect the position of the cover glass–microlens junction in the z -direction ( Fig. 3 ). Once the CaCO 3 microlens arrays are transferred from the solution within 1–3 h and dried, the amorphous phase is kept up to several months in ambient atmosphere depending on the humidity. Indeed, ACC synthesized in high pH precursor solution (in this study pH 12.5) has been reported to be more stable than that formed at a lower pH [39] . When the growth of the CaCO 3 microlens array proceeds for more than 4 h at the air–Ca(OH) 2 solution interface, some structures are protruded on the convex surface of microlenses, which further grow into (104) faceted crystals ( Supplementary Fig. S8 ) [40] . Cell culture on microlens array The microlens array–coated cover slides were sterilized under ultraviolet light for 1 h, and NIH3T3 fibroblasts were seeded and cultured overnight in DMEM medium (Sigma) with 10% calf serum at 37 °C inside an incubator under humidified atmosphere. Later, microlens arrays were washed a few times in PBS, and the cells were fixed in 4% paraformaldehyde (Fluka) for 5 min at room temperature. Unbound paraformaldehyde was removed by gentle washing in PBS several times. Cells were permeabilized with 0.1% Triton X-100 (Sigma) for 5 min and stained with 1:200 diluted Alexa Fluor 488 (Invitrogen) for 60 min. Nucleus staining was performed with 1:300 diluted TOPRO-3 Iodide (Invitrogen) for 5 min and the microlens array cover slides were washed in PBS, mounted with Vectashield mounting medium and observed under confocal laser scanning microscope (Leica TCS SP5, Leica). Characterization of the focal length The experiment has been performed on a laser scanning confocal microscope (Leica DM IRBE, Leica) in two steps, as depicted in Supplementary Fig. S9 . First, 488-nm laser light was focused on the sample using a microscope objective (oil ×100, 1.4 NA, Leica) and scanned across the field of view. The fluorescence was collected by the objective (epifluorescence mode) and detected by a photomultiplier tube (PMT) through a dichroic mirror (RSP 500, Leica). The signal was spectrally selected by a monochromator set to collect wavelengths between 505 and 560 nm. One image contained 1,024×1,024 pixels and a final image was created by an average of four recorded images. The sample was scanned at decreasing height by steps of 0.2 μm. A total of 80 images was recorded and used to generate a stack of 16 μm in depth. Second, a laser pointer (640–660 nm, Hama laserpointer LP-18, Hama) was secured above the microscope stage using a laboratory buret stand and an extension clamp. The collimated light was directed perpendicular to the coverslip slide supporting the microlens array and collected by the microscope objective. Alignment of the laser beam was adjusted by reflection of part of the light by the microscope slide surface supporting the sample. The monochromator was set to select light between 630 and 670 nm, and an image stack was generated as described above. Characterization methods The surface tension measurement was carried out using a DuNouy Tensionmeter (KRÜSS Tensionmeter K12). The projected images of 'A' through the CaCO 3 microlens arrays were obtained by using optical microscopy (Leica DM RXA2, Leica; fitted with a digital colour camera, Leica DFC 480, Leica) set with microlens array and screen 'A' on the object stage in transmission mode. For confocal Raman microspectroscopy (WITec alpha300R, WITec), the selected area of the sample was scanned with a continuous green laser beam with lateral and depth resolutions of 250 and 500 nm, respectively. Raman images have been generated by integrating the intensity of the signal for the wavenumber ranges of carbonate (1,040~1,125 cm −1 , Fig. 3a ), water (3,000~3,500 cm −1 , Fig. 3b ) and organic (2,800~3,000 cm −1 , Fig. 3c ). How to cite this article: Lee, K. et al . Self-assembly of amorphous calcium carbonate microlens arrays. Nat. Commun. 3:725 doi: 10.1038/ncomms1720 (2012).